RhoB controls coordination of adult angiogenesis and lymphangiogenesis following injury by regulating VEZF1-mediated transcription Mechanisms governing the distinct temporal dynamics that characterize post-natal angiogenesis and lymphangiogenesis elicited by cutaneous wounds and inflammation remain unclear. RhoB, a stress-induced small GTPase, modulates cellular responses to growth factors, genotoxic stress and neoplastic transformation. Here we show, using RhoB null mice, that loss of RhoB decreases pathological angiogenesis in the ischaemic retina and reduces angiogenesis in response to cutaneous wounding, but enhances lymphangiogenesis following both dermal wounding and inflammatory challenge. We link these unique and opposing roles of RhoB in blood versus lymphatic vasculatures to the RhoB-mediated differential regulation of sprouting and proliferation in primary human blood versus lymphatic endothelial cells. We demonstrate that nuclear RhoB-GTP controls expression of distinct gene sets in each endothelial lineage by regulating VEZF1-mediated transcription. Finally, we identify a small-molecule inhibitor of VEZF1–DNA interaction that recapitulates RhoB loss in ischaemic retinopathy. Our findings establish the first intra-endothelial molecular pathway governing the phased response of angiogenesis and lymphangiogenesis following injury. Large organisms exhibit two different vascular networks essential for life. The circulatory blood vascular network, arising during embryonic development by both vasculogenesis and angiogenesis, provides oxygen, nutrients, hormones and cells to tissues, and collects carbon dioxide and other metabolic waste products [1] . The blind-ended lymphatic vascular network that subsequently originates from the embryonic cardinal vein by budding and differentiation of a subpopulation of blood vascular endothelial cells (BVECs) regulates tissue fluid homoeostasis, immune cell trafficking and absorption of dietary fats [2] . Similarly in adults, studies have shown that angiogenesis precedes lymphangiogenesis during the repair of damaged tissues [3] , [4] , [5] , [6] , [7] , [8] , [9] . However, the underlying mechanisms that timely coordinate these processes are still elusive. Considering the close identity between blood and lymphatic endothelial cells, a central question still unresolved is how blood vessels quickly engage in the revascularization of damaged tissues, while the growth of lymphatics is delayed in response to the same pathological stimulus. RhoB is an immediate early response gene rapidly inducible by many stimuli including genotoxic stress, cytokines and growth factors [10] , [11] , [12] , [13] . In contrast to related members of the RhoA/Rac1/Cdc42 family of small GTPases, RhoB is primarily localized on endosomes and in the nucleus, and has been shown to regulate vesicle and growth factor receptor trafficking [14] , [15] , [16] , [17] , [18] . RhoB null mice are viable, indicating that RhoB is dispensable for normal development [19] ; however, RhoB can alter tumour formation by limiting tumour cell growth but yet promoting tumour angiogenesis [20] , [21] . Studies in RhoB null mice indicate that RhoB is a critical modifier of apoptosis triggered by genotoxic stress. RhoB promotes apoptosis in response to DNA damage in transformed fibroblasts [19] , but protects transformed keratinocytes from UVB-induced apoptosis, suggesting that RhoB’s functions are both stress- and context-dependent [13] . Our previous studies revealed the contribution of this small GTPase to the blood vasculature in the developing retina, that is, defective endothelial tip cell sprouting occurred in RhoB null mice [18] . We found that RhoB is a determinant of Akt stability and trafficking to the nucleus, and that this function has a stage-specific role in the survival of sprouting BVECs that contribute to new blood vessel assembly during post-natal retinal development. Given its critical roles in both the stress response and vascular morphogenesis, we hypothesized that RhoB might also be relevant in adult pathological scenarios involving endothelial cell challenge, such as wound healing, inflammation or reperfusion injury. Herein we examine the effect of RhoB deletion on pathological angiogenesis associated with ischaemic retinopathy, as well as on angiogenesis and lymphangiogenesis elicited by dermal injury or inflammation. Using primary human BVECs versus lymphatic vascular endothelial cells (LVECs), we investigate the role that RhoB serves in regulating proliferation and sprouting in these two endothelial populations. We explore the possibility that RhoB is functionally linked to the zinc finger transcription factor DB1/VEZF1, a molecule known to regulate embryonic angiogenesis and lymphangiogenesis [22] , and previously reported to be a RhoB-interacting protein in vitro [14] . We perform transcriptome analyses to uncover unique sets of relevant genes targeted by VEZF1 and co-regulated by RhoB in BVECS versus LVECs, leading us to postulate a novel mechanism responsible for the temporally coordinated response of the blood and lymphatic networks to injury. RhoB loss normalizes blood vasculature in OIR We employed the mouse model of oxygen-induced retinopathy (OIR) [23] in neonatal wild-type ( wt ) and RhoB −/− mice to evaluate the effect of RhoB loss in a pathological angiogenic environment. After 5 days at 70% oxygen (P7–P12), the retinal vasculature in both wt and RhoB −/− pups exhibited profound vessel regression, particularly in the central portion near the optic disc (OD), confirming that the initial vascular response to high oxygen is not altered in the absence of RhoB ( Fig. 1a , Supplementary Fig. S1 ). Subsequently, after 5 days of room air (P12–P17), wt pups mounted a robust pathological neovascularization typified by abnormalities in vascular structure, that is, formation of glomeruloid bodies or ‘vascular tufts’ (arrowheads), large avascular areas (star) and endothelial cell invasion through the inner limiting membrane (ILM) into the vitreous (arrows). In contrast, RhoB −/− mice showed a dramatic reduction in glomeruloid bodies and 100-fold reduced intra-vitreous invasion rate. RhoB loss during ischaemic retinal neovascularization converts the resultant pathological neovascular network to a more physiological phenotype. 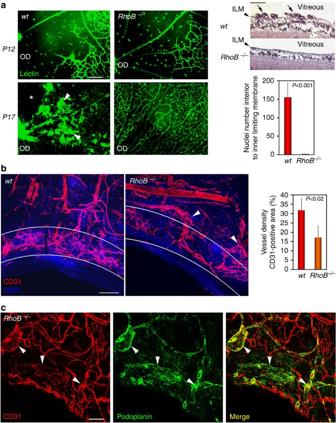Figure 1: RhoB loss normalizes angiogenesis in OIR and decreases BV density in granulation tissue. (a) Whole-mount staining of blood vessels (BS-I lectin) in the retina ofwtandRhoB−/−pups subjected to hyperoxia from P7 to P12, and then returned back to normoxia from P12 to P17 (OD, optic disc). Histological (H&E) analysis ofwtandRhoB−/−retinas at P17. Quantification of nuclei number interior to ILM (n=10 mice per genotype, mean±s.e.m., unpaired two-tailed Student’st-test). (b) Confocal analysis following whole-mount staining of CD31 expression in the granulation tissue present 7 days after ear wounding in adultwtandRhoB−/−mice (6–8 weeks old). Quantification of CD31-positive staining in the neovasculature of the granulation tissue (delineated with white lines) (n=6 mice per genotype, mean±s.e.m., unpaired two-tailed Student’st-test). (c) Confocal analysis following whole-mount staining of CD31 and podoplanin expression in the granulation tissue present 7 days after wounding. Arrowheads highlight lymphatic vessels and denote areas of colocalization of CD31 and podoplanin in the merged image, thus confirming the identity of the lymphatic vessels. Scale bars: whole-mount staining=100 μm, H&E sections=50 μm (a), 200 μm (b,c). Figure 1: RhoB loss normalizes angiogenesis in OIR and decreases BV density in granulation tissue. ( a ) Whole-mount staining of blood vessels (BS-I lectin) in the retina of wt and RhoB −/− pups subjected to hyperoxia from P7 to P12, and then returned back to normoxia from P12 to P17 (OD, optic disc). Histological (H&E) analysis of wt and RhoB −/− retinas at P17. Quantification of nuclei number interior to ILM ( n =10 mice per genotype, mean±s.e.m., unpaired two-tailed Student’s t -test). ( b ) Confocal analysis following whole-mount staining of CD31 expression in the granulation tissue present 7 days after ear wounding in adult wt and RhoB −/− mice (6–8 weeks old). Quantification of CD31-positive staining in the neovasculature of the granulation tissue (delineated with white lines) ( n =6 mice per genotype, mean±s.e.m., unpaired two-tailed Student’s t -test). ( c ) Confocal analysis following whole-mount staining of CD31 and podoplanin expression in the granulation tissue present 7 days after wounding. Arrowheads highlight lymphatic vessels and denote areas of colocalization of CD31 and podoplanin in the merged image, thus confirming the identity of the lymphatic vessels. Scale bars: whole-mount staining=100 μm, H&E sections=50 μm ( a ), 200 μm ( b , c ). Full size image Angiogenesis and lymphangiogenesis in RhoB −/− wounds To evaluate the impact of RhoB deletion in another tissue, we subjected the mouse ear to a full-thickness wound. New blood vessels appeared in the granulation tissue of wt mice by day 7 after wounding ( Fig. 1b ), whereas after 1 week RhoB −/− mice exhibited poor neovascularization with a twofold decreased vascular density. Interestingly in RhoB −/− mice, CD31 immunostaining revealed not only the presence of positively stained blood vessels, but additional structures with a different morphology and weak staining intensity (arrowheads). CD31 is also known to be expressed by lymphatic endothelial cells [24] . To validate the lymphatic identity of these additional vascular structures, we stained for podoplanin, a protein that is specifically expressed in the lymphatic endothelium ( Fig. 1c ). Colocalization of CD31 and podoplanin confirmed numerous lymphatic vessels infiltrating and surrounding the granulation tissue specifically in RhoB −/− mice (arrowheads). In agreement with previous studies [6] , [9] , [25] , injection of macromolecular FITC–dextran tracer into the dermal lymphatic vessels in wt mice on day 7 post-wounding revealed no obvious new lymphatics associated with the granulation tissue ( Fig. 2a and Supplementary Movie 1 ). In contrast, RhoB −/− mice exhibited a profound lymphangiogenic response as judged by the rapid filling of a distinct lymphatic network beginning between 2–10 s after tracer injection and progressively increasing by 30 s ( Supplementary Movie 2 ), indicating more numerous lymphatic vessels (twofold increase) and an elevated interconnectivity in the lymphatic network adjacent to the wound. Thereafter, between 30 and 60 s, FITC–dextran accumulated in the tissue immediately surrounding the filled lymphatics (arrowheads), far from the tracer injection site, suggesting an abnormal structure of these new lymphatics leading to the enhanced leakage of fluid and macromolecules. Confocal analysis following whole-mount staining with anti-podoplanin confirmed lymphatic lumen enlargement and impaired lymphatic barrier integrity in the RhoB −/− granulation tissue (respectively, arrowhead and star, Fig. 2b ). 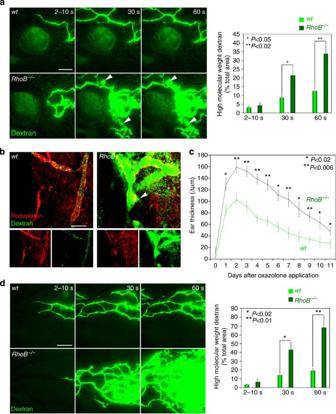Figure 2: RhoB loss leads to enhanced and abnormal lymphangiogenesis in response to stress. (a) Intravital microlymphangiography byin vivoinjection of FITC–dextran (MW 2,000 kDa) into lymphatics of ear skin 7 days after ear wounding in adultwtandRhoB−/−mice. Dextran-positive areas in isolated frames taken from the movies at early (2–10 s (s)), middle (30 s) and late (60 s) times following tracer injection were quantified (n=7 mice per genotype, mean±s.e.m., unpaired two-tailed Student’st-test). (b) Confocal analysis followingin vivoFITC–dextran injection in lymphatics and whole-mount staining of podoplanin expression in the granulation tissue present 7 days after ear wounding in adultwtandRhoB−/−mice. Arrowhead and star respectively highlight dextran leakage from an abnormal lymphatic vessel and tracer accumulation in the adjacent tissue ofRhoB−/−mice in the merged image. (c) Induction of DTH reactions in the ear skin of adultwtandRhoB−/−mice. Ear swelling is expressed as the increase (Δ) over the original ear thickness in μm. Ear thickness was measured daily for 11 days following challenge using a Mitutoyo caliper (n=12 mice per genotype, mean±s.e.m., unpaired two-tailed Student’st-test). (d) Intravital microlymphangiography byin vivoinjection of FITC–dextran (MW 2,000 kDa) into lymphatics of ear skin 7 days after inflammation induced by oxazolone in adultwtandRhoB−/−mice. FITC–dextran-positive areas in isolated frames taken from movies at early (2–10 s (s)), middle (30 s) and late (60 s) times following tracer injection were quantified (n=6 mice per genotype, mean±s.e.m., unpaired two-tailed Student’st-test). Scale bars: 1 mm (a,d) and 100 μm (b). Figure 2: RhoB loss leads to enhanced and abnormal lymphangiogenesis in response to stress. ( a ) Intravital microlymphangiography by in vivo injection of FITC–dextran (MW 2,000 kDa) into lymphatics of ear skin 7 days after ear wounding in adult wt and RhoB −/− mice. Dextran-positive areas in isolated frames taken from the movies at early (2–10 s (s)), middle (30 s) and late (60 s) times following tracer injection were quantified ( n =7 mice per genotype, mean±s.e.m., unpaired two-tailed Student’s t -test). ( b ) Confocal analysis following in vivo FITC–dextran injection in lymphatics and whole-mount staining of podoplanin expression in the granulation tissue present 7 days after ear wounding in adult wt and RhoB −/− mice. Arrowhead and star respectively highlight dextran leakage from an abnormal lymphatic vessel and tracer accumulation in the adjacent tissue of RhoB −/− mice in the merged image. ( c ) Induction of DTH reactions in the ear skin of adult wt and RhoB −/− mice. Ear swelling is expressed as the increase (Δ) over the original ear thickness in μm. Ear thickness was measured daily for 11 days following challenge using a Mitutoyo caliper ( n =12 mice per genotype, mean±s.e.m., unpaired two-tailed Student’s t -test). ( d ) Intravital microlymphangiography by in vivo injection of FITC–dextran (MW 2,000 kDa) into lymphatics of ear skin 7 days after inflammation induced by oxazolone in adult wt and RhoB −/− mice. FITC–dextran-positive areas in isolated frames taken from movies at early (2–10 s (s)), middle (30 s) and late (60 s) times following tracer injection were quantified ( n =6 mice per genotype, mean±s.e.m., unpaired two-tailed Student’s t -test). Scale bars: 1 mm ( a , d ) and 100 μm ( b ). Full size image RhoB loss enhances lymphangiogenesis in chronic inflammation Using oxazolone as a sensitizing agent [26] , we induced a delayed-type hypersensitivity (DTH) reaction and assessed the level of oedema accompanying this model of chronic inflammation by measurement of ear thickness ( Fig. 2c ). The maximum extent of oedema, reached by day 2 after oxazolone application, was significantly higher in RhoB −/− ears as compared to wt . Thereafter, ear swelling declined more slowly and remained significantly higher in RhoB −/− compared with wt mice even after 11 days, indicating that resolution of fluids that accumulated during the inflammatory phase is impaired in the RhoB −/− mice. Visualization of the lymphatic network at 7 days post challenge by intralymphatic injection of FITC–dextran tracer revealed a massive lymphangiogenic response in RhoB −/− mice characterized by more numerous lymphatic vessels, enhanced lymphatic interconnectivity and dramatic FITC–dextran leakage into the surrounding tissue ( Fig. 2d , Supplementary Movie 4 ) as compared with wt ( Supplementary Movie 3 ). RhoB differentially affects BVEC and LVEC response to stress Using pure populations of human primary BVECs and LVECs isolated from foreskin ( Supplementary Fig. S2 ), we determined the relative amounts of RhoB protein found in BVECs versus LVECs during resting conditions (cells at 100% confluence for 48 h without media renewal), or during proliferative conditions (cells collected 24 h and 48 h after challenge initiated by trypsinization of confluent cultures followed by re-plating at 50% density) ( Fig. 3a ). RhoB was constitutively expressed in both resting and proliferating BVECs, but was barely detectable in LVECs at rest and at 48 h after challenge. Interestingly, the level of RhoB protein increased in both BVECs and LVECs 24 h after proliferative challenge, suggesting that RhoB has a critical role in the immediate response of both BVECs and LVECs to stress. Next, we either silenced or overexpressed RhoB , by siRNA nucleofection or adenovirus infection, respectively, and subjected confluent cultures of the modified cells to proliferative stress ( Fig. 3b ). Immunostaining of pre-confluent cells 24 h following proliferative stress for the proliferation marker Ki67 showed that RhoB silencing decreased the percent of proliferating BVECs twofold, but nearly doubled the percent of proliferating of LVECs ( Fig. 3c ). In direct contrast, RhoB overexpression significantly promoted the proliferation of BVECs, but repressed LVECs proliferation. Finally, using a three-dimensional (3D) sprouting assay, we observed that RhoB silencing reduced the sprouting of BVECs induced by VEGF-A and led to increased sprouting of LVECs stimulated by VEGF-C ( Fig. 3d ). In contrast, RhoB overexpression had the reverse effect, that is, a higher number of BVECs sprouted in response to VEGF-A, and a lower number of LVECs sprouted in response to VEGF-C ( Fig. 3d ). These results demonstrate that RhoB serves cell-autonomous, yet opposing, roles in two essential features of blood and lymphatic endothelial cell biology, that is, proliferation and sprouting. Overall these in vitro results equate directly with our in vivo observations: (1) in the OIR model, the dramatic reduction in the number of glomeruloid bodies, which are formed as a consequence of BVEC hyper-proliferation in the retina and (2) in the dermal wound healing and DTH models, the enlarged, highly interconnected and leaky lymphatic vessels, which were previously shown to be correlated with LVEC proliferation and the unstable sprouting tip cell phenotype [27] , [28] , [29] . 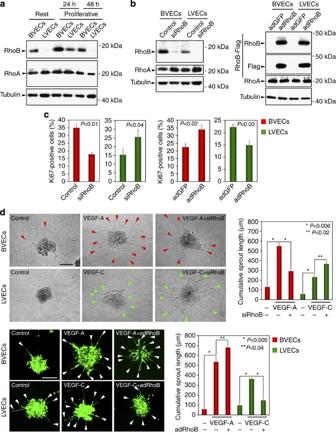Figure 3: Differential regulation of proliferation and sprouting in BVECs and LVECs by RhoB. (a) Representative western blot showing the endogenous level of RhoB protein in BVECs and LVECs in the resting state (100% confluence for 48 h without media renewal) versus the proliferative state (24 h and 48 h after challenge initiated by cell plating at low, that is, 50%, density). Western blotting for a related GTPase, RhoA, did not indicate any variation in RhoA expression levels in BVECs or LVECs under resting or proliferative conditions and thus confirmed the specificity of the RhoB antibody and the unique regulation ofRhoBin these cells. Tubulin was used as loading control. (b) Representative western blot showing the efficiency ofRhoBsilencing by siRNA nucleofection, and the level ofRhoBoverexpression following adenovirus infection, in BVECs and LVECs 24 h after proliferative challenge. The RhoB-Flag protein was detected using antibodies directed against the RhoB protein and by antibodies against the Flag tag. (c) Proliferation index of BVECs and LVECs afterRhoBsilencing andRhoBoverexpression at 24 h after proliferative challenge, determined as the ratio of the number of Ki67 positive cells to the total number of cells (expressed as %,n≥600 total cells taken from at least six fields with at least 100 cells per field per condition, mean±s.e.m., unpaired two-tailed Student’st-test). (d) Sprouting from BVECs and LVECs spheroids in 3D Matrigel–collagen I matrix, induced for 24 h by VEGF-A or VEGF-C, respectively, afterRhoBsilencing (phase-contrast pictures) orRhoBoverexpression (fluorescent confocal projections). GFP expression, resulting from infection with the RhoB adenoviral vector containing an IRES-GFP, was used as an internal control for the overexpression experiments. Individual sprouts inRhoB-silenced cells are noted by red (BVECs) or green (LVECs) arrowheads, and inRhoB-overexpressing cells by white arrowheads. Quantitative analysis of endothelial cell sprouting was performed by measuring the cumulative length of all of the sprouts originating from one spheroid (described previously47), using NIH ImageJ software (n=10 spheroids, mean±s.e.m., unpaired two-tailed Student’st-test). Scale bars: 50 μm (d). Figure 3: Differential regulation of proliferation and sprouting in BVECs and LVECs by RhoB. ( a ) Representative western blot showing the endogenous level of RhoB protein in BVECs and LVECs in the resting state (100% confluence for 48 h without media renewal) versus the proliferative state (24 h and 48 h after challenge initiated by cell plating at low, that is, 50%, density). Western blotting for a related GTPase, RhoA, did not indicate any variation in RhoA expression levels in BVECs or LVECs under resting or proliferative conditions and thus confirmed the specificity of the RhoB antibody and the unique regulation of RhoB in these cells. Tubulin was used as loading control. ( b ) Representative western blot showing the efficiency of RhoB silencing by siRNA nucleofection, and the level of RhoB overexpression following adenovirus infection, in BVECs and LVECs 24 h after proliferative challenge. The RhoB-Flag protein was detected using antibodies directed against the RhoB protein and by antibodies against the Flag tag. ( c ) Proliferation index of BVECs and LVECs after RhoB silencing and RhoB overexpression at 24 h after proliferative challenge, determined as the ratio of the number of Ki67 positive cells to the total number of cells (expressed as %, n ≥600 total cells taken from at least six fields with at least 100 cells per field per condition, mean±s.e.m., unpaired two-tailed Student’s t -test). ( d ) Sprouting from BVECs and LVECs spheroids in 3D Matrigel–collagen I matrix, induced for 24 h by VEGF-A or VEGF-C, respectively, after RhoB silencing (phase-contrast pictures) or RhoB overexpression (fluorescent confocal projections). GFP expression, resulting from infection with the RhoB adenoviral vector containing an IRES-GFP, was used as an internal control for the overexpression experiments. Individual sprouts in RhoB -silenced cells are noted by red (BVECs) or green (LVECs) arrowheads, and in RhoB -overexpressing cells by white arrowheads. Quantitative analysis of endothelial cell sprouting was performed by measuring the cumulative length of all of the sprouts originating from one spheroid (described previously [47] ), using NIH ImageJ software ( n =10 spheroids, mean±s.e.m., unpaired two-tailed Student’s t -test). Scale bars: 50 μm ( d ). Full size image RhoB collaborates with VEZF1 To decipher the molecular mechanisms responsible for the differential effect of RhoB in blood and lymphatic vascular beds, we investigated the possibility that RhoB is functionally linked to the zinc finger transcription factor VEZF1. VEZF1 is known to regulate embryonic angiogenesis and lymphangiogenesis [22] , and has previously been reported to be a RhoB-interacting protein in vitro [14] . As VEZF1 −/− mice are embryonic lethal, we crossed mice from the RhoB and VEZF1 heterozygotes and generated an allelic series of mice, that is, RhoB +/− , VEZF1 +/− and RhoB +/− VEZF1 +/− . Using the OIR assay, we observed that loss of only one RhoB allele did not alter the pathological angiogenic response in the retina of RhoB +/− mice as compared with wt ( Fig. 4a ). However, VEZF1 +/− mice exhibited a reduced pathological angiogenic response (twofold decrease in the number of nuclei interior to ILM) ( Fig. 4a ), which is further reprogrammed to more physiological angiogenesis in RhoB +/− VEZF1 +/− mice, similarly to RhoB −/− mice ( Fig. 4a ). In parallel, we assessed the lymphangiogenic response to challenge using the ear wound model. By day 7 post wounding, in dramatic contrast to what we observed in the RhoB −/− mice ( Fig. 2a ), injection of FITC–dextran tracer did not reveal new lymphatics in the region immediately surrounding the site of the wound in RhoB +/− mice ( Fig. 4b and Supplementary Movie 5 ). In contrast, in RhoB +/− VEZF1 +/− mice, the lymphangiogenic response was comparable to that observed in the RhoB −/− mice ( Fig. 4b and Supplementary Movie 7 ). Interestingly, VEZF1 +/− mice exhibit an intermediate lymphatic phenotype with the emergence of several leaky lymphatics around the granulation tissue (arrowhead, Fig. 4b , Supplementary Movie 6 ). 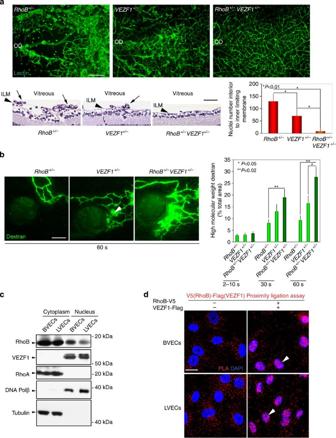Figure 4: Functional interaction between RhoB and VEZF1 during OIR and wound healing. (a) Whole-mount staining of blood vessels (BS-I lectin) in the retina ofRhoB+/−,VEZF1+/−andRhoB+/−VEZF1+/−pups (P17) subjected to OIR assay (OD=Optic Disc). Histological (H&E) analysis ofRhoB+/−,VEZF1+/−andRhoB+/−VEZF1+/−retinas at P17. Quantification of the number of nuclei interior to ILM (n=6 per genotype, mean±s.e.m., unpaired two-tailed Student’st-test). (b) Intravital microlymphangiography byin vivoinjection of FITC–dextran (MW 2,000 kDa) into lymphatics of ear skin 7 days after ear wounding in adultRhoB+/−,VEZF1+/−andRhoB+/−VEZF1+/−mice, shown at 60 s post tracer injection. Dextran-positive areas in isolated frames taken from the movies at early (2–10 s (s)), middle (30 s) and late (60 s) times following tracer injection were quantified (n=6 mice per genotype, mean±s.e.m., unpaired two-tailed Student’st-test). (c) Representative western blot of nuclear and cytoplasmic extracts showing the dual localization of RhoB in both nuclei and cytoplasm of BVECs and LVECs, whereas another RhoGTPase, RhoA, was detected only in the cytoplasm. In contrast, VEZF1 was exclusively detected in nuclei. DNA Polβ and Tubulin proteins were used as internal controls for nuclear and cytoplasmic extracts, respectively. (d) Confocal analysis ofin situproximity ligation assay (PLA) (red) using anti-V5 and anti-Flag allows visualization of the interaction of RhoB-V5 and VEZF1-Flag in the nucleus (DAPI—blue) of both transfected BVECs and LVECs (right panels—arrowheads) versus control untransfected cells (left panels), which exhibit only non-specific background staining in the cytoplasm. Scale bars: whole-mount staining=100 μm, H&E sections=50 μm (a), 1 mm (b) and 10 μm (d). Figure 4: Functional interaction between RhoB and VEZF1 during OIR and wound healing. ( a ) Whole-mount staining of blood vessels (BS-I lectin) in the retina of RhoB +/− , VEZF1 +/− and RhoB +/− VEZF1 +/− pups (P17) subjected to OIR assay (OD=Optic Disc). Histological (H&E) analysis of RhoB +/− , VEZF1 +/− and RhoB +/− VEZF1 +/− retinas at P17. Quantification of the number of nuclei interior to ILM ( n =6 per genotype, mean±s.e.m., unpaired two-tailed Student’s t -test). ( b ) Intravital microlymphangiography by in vivo injection of FITC–dextran (MW 2,000 kDa) into lymphatics of ear skin 7 days after ear wounding in adult RhoB +/− , VEZF1 +/− and RhoB +/− VEZF1 +/− mice, shown at 60 s post tracer injection. Dextran-positive areas in isolated frames taken from the movies at early (2–10 s (s)), middle (30 s) and late (60 s) times following tracer injection were quantified ( n =6 mice per genotype, mean±s.e.m., unpaired two-tailed Student’s t -test). ( c ) Representative western blot of nuclear and cytoplasmic extracts showing the dual localization of RhoB in both nuclei and cytoplasm of BVECs and LVECs, whereas another RhoGTPase, RhoA, was detected only in the cytoplasm. In contrast, VEZF1 was exclusively detected in nuclei. DNA Polβ and Tubulin proteins were used as internal controls for nuclear and cytoplasmic extracts, respectively. ( d ) Confocal analysis of in situ proximity ligation assay (PLA) (red) using anti-V5 and anti-Flag allows visualization of the interaction of RhoB-V5 and VEZF1-Flag in the nucleus (DAPI—blue) of both transfected BVECs and LVECs (right panels—arrowheads) versus control untransfected cells (left panels), which exhibit only non-specific background staining in the cytoplasm. Scale bars: whole-mount staining=100 μm, H&E sections=50 μm ( a ), 1 mm ( b ) and 10 μm ( d ). Full size image To address the interaction of RhoB with VEZF1 at the molecular level, we investigated the subcellular localization of these two proteins in BVECs and LVECs. Although RhoB was detected predominantly in the cytoplasm of both BVECs and LVECs, in both cell types this small GTPase was also located in the nucleus, where VEZF1 protein was exclusively detected ( Fig. 4c ). Moreover, using a proximity ligation assay we were able to demonstrate a protein complex containing V5-tagged RhoB and Flag-tagged VEZF1 located in the nucleus of both BVECs and LVECs ( Fig. 4d , arrowheads). Taken together, these studies strongly argue that RhoB genetically interacts with VEZF1 in the regulation of the altered blood vascular response to ischaemia as well as in the temporal repression of lymphangiogenesis during wound healing, and indicate that RhoB belongs to a nuclear transcriptional complex containing VEZF1. RhoB and VEZF1 share target genes in BVECs and LVECs To uncover how the collaboration between RhoB and VEZF1 affects BVEC and LVEC biology, we performed Affymetrix microarray analyses after silencing either RhoB or VEZF1 in both endothelial cell types ( Supplementary Fig. S3 ). A significant number of the deregulated probe sets in RhoB -silenced BVECs matched the deregulated probe sets in VEZF1 -silenced BVECs (214 downregulated and 243 upregulated probe sets). Similarly, 1,413 downregulated probe and 1,280 upregulated probe sets in RhoB -silenced LVECs compared favourably to the deregulated probe sets in VEZF1 -silenced LVECs, suggesting that these deregulated probe sets could correspond to the specific genes targeted by VEZF1 and co-regulated by RhoB. Using gene ontology (GO) classification to query the function of the target genes shared by RhoB and VEZF1, we identified ontology categories important for different aspects of endothelial cell biology including proliferation and sprouting ( Supplementary Table S1 ). Among the subsets of shared target genes ( Supplementary data 1 ), we confirmed the role of RhoB and VEZF1 in the regulation of expression of a finite number of particularly relevant genes by QRT–PCR ( Fig. 5a , Supplementary Fig. S4a ). For example, the VEGF-A receptor, VEGF-R2, and its co-receptor, Neuropilin1 (NRP1), were both downregulated in BVECs after silencing of either RhoB or VEZF1 (twofold decrease in silenced cells compared with control). Although these two genes were also detected in the LVECs microarrays, QRT–PCRs revealed a lower basal level of expression and an insignificant decrease after silencing of either RhoB or VEZF1 in these cells, suggesting a predominant effect of RhoB-VEZF1 on VEGF-R2 and NRP1 expression in BVECs compared with that in LVECs. By contrast, the metallopeptidase inhibitor, TIMP3, was more highly expressed in LVECs, suggesting that downregulation of this protein, triggered by both RhoB and VEZF1 knockdown, has a particularly potent impact in LVECs versus BVECs. 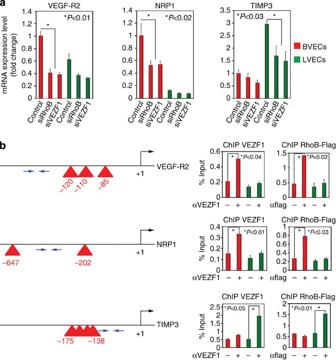Figure 5: Target genes shared by RhoB and VEZF1 in BVECs and LVECs. (a) Relative mRNA levels of VEGF-R2, NRP1 and TIMP3 in BVECs and LVECs following silencing of either RhoB or VEZF1 as determined by QRT–PCR (performed in triplicate on two different cell isolation lots, mean±s.e.m., unpaired two-tailed Student’st-test). (b)In vivobinding of VEZF1 and RhoB-Flag to the promoter region of target genes, that is, VEGF-R2, NRP1 and TIMP3, containing predictedin silicoVEZF1 DNA binding sites (red triangle in schematic drawing of promoters) assessed by ChIP experiments. The start site of transcription is referred as +1. The position of primers used for QRT–PCR experiments is represented by blue arrows. The enrichment for each DNA fragment upon immunoprecipitation of VEZF1 and RhoB-Flag is illustrated as histograms based on % of input (QRT–PCR performed in triplicate on two different cell isolation lots, mean±s.e.m., unpaired two-tailed Student’st-test). Figure 5: Target genes shared by RhoB and VEZF1 in BVECs and LVECs. ( a ) Relative mRNA levels of VEGF-R2, NRP1 and TIMP3 in BVECs and LVECs following silencing of either RhoB or VEZF1 as determined by QRT–PCR (performed in triplicate on two different cell isolation lots, mean±s.e.m., unpaired two-tailed Student’s t -test). ( b ) In vivo binding of VEZF1 and RhoB-Flag to the promoter region of target genes, that is, VEGF-R2, NRP1 and TIMP3, containing predicted in silico VEZF1 DNA binding sites (red triangle in schematic drawing of promoters) assessed by ChIP experiments. The start site of transcription is referred as +1. The position of primers used for QRT–PCR experiments is represented by blue arrows. The enrichment for each DNA fragment upon immunoprecipitation of VEZF1 and RhoB-Flag is illustrated as histograms based on % of input (QRT–PCR performed in triplicate on two different cell isolation lots, mean±s.e.m., unpaired two-tailed Student’s t -test). Full size image To identify the direct target genes of VEZF1, and more importantly, those that are also co-regulated by RhoB, we analysed the binding of these two proteins to a number of selected promoters by chromatin immunoprecipitation (ChIP). Initially, we confirmed chromatin enrichment of the endothelin1 promoter, known to be a direct target of VEZF1 (ref. 30 ), in BVECS after VEZF1 immunoprecipitation, thus validating our ChIP protocol ( Supplementary Fig. S4b ). Interestingly, we also discovered sequences containing potential VEZF1 DNA binding sites in the promoter regions of VEGF-R2 and NRP1 ( Fig. 5b ). These regions exhibit three- and twofold enrichment, respectively, after VEZF1 or RhoB-Flag immunoprecipitation, specifically in BVECs. In contrast, the chromatin of the TIMP3 promoter regions, which also contains putative VEZF1 DNA binding sites, is enriched fourfold after VEZF1 or RhoB-Flag immunoprecipitation, specifically in LVECs ( Fig. 5b ). Taken together, these data suggest that RhoB works in conjunction with VEZF1 on specific promoters to regulate the expression of essential direct target genes involved in the proliferation and sprouting of endothelial cells. Of critical importance, these sets of direct targets appear to be different in BVECs versus LVECs. RhoB-GTP specifically controls BVEC and LVEC proliferation A significant feature of many small GTPases is their ability to toggle intrinsic GTPase activity between ‘on’ and ‘off’ states, as determined by the ratio of the GTP-bound to the GDP-bound forms of the enzyme [31] . To assess the importance of these two states in the regulatory function of RhoB in endothelial cells, we prepared adenoviral vectors encoding mutants of RhoB and used them to elicit overexpression of three different forms of the RhoB GTPase: wt (adRhoB), the RhoB dominant negative form corresponding to the GDP-bound state (adRhoB-DN) and the RhoB constitutively active form corresponding to the GTP-bound state (adRhoB-CA). Overexpression of wt or mutant RhoB was performed in BVECs and LVECs undergoing proliferative challenge and the corresponding GTP levels were measured by GTP pull-down assay ( Fig. 6a ). Neither BVECs nor LVECs infected with adRhoB-DN exhibited any detectable amount of GTP-bound RhoB, whereas both cell types infected with adRhoB-CA showed high levels of expression of the GTP-bound form of RhoB. Following wt RhoB overexpression, a substantial amount of RhoB in the GTP-bound state could be detected in both BVECs and LVECs, indicating that both cell types maintain RhoB in a predominantly active form under proliferating conditions. To evaluate the possibility that the state of RhoB determines its localization within the cell, we analysed the subcellular pattern of these RhoB mutants ( Fig. 6b ). wt RhoB and all mutants of RhoB, including the dominant negative RhoB, were detected in the cytoplasm as well as in the nucleus of BVECs and LVECs, indicating that both the GTP- and the GDP-bound states of RhoB can be found within the nucleus. 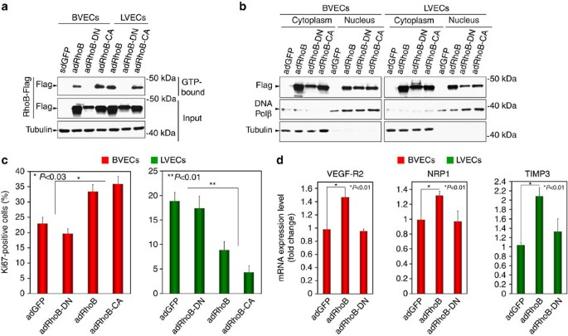Figure 6: BVEC and LVEC proliferation is specifically regulated by GTP-bound state of RhoB. (a) Representative western blot for detection of RhoB protein activation by GTP pull-down assay after adenoviral-mediated overexpression of wt RhoB-Flag (adRhoB) and RhoB mutants, that is, adRhoB-DN for dominant negative (GDP-bound state), adRhoB-CA for constitutive active (GTP-bound state). AdGFP was used as the control. Anti-RhoB and anti-Flag antibodies successfully detected all RhoB-Flag proteins in input samples. (b) Representative western blot of nuclear and cytoplasmic extracts from BVECs and LVECs showing the dual localization of overexpressed wt RhoB-Flag and its mutants in both nuclei and cytoplasm of BVECs and LVECs. AdGFP was used as the control. DNA Polβ and Tubulin proteins were used as internal controls for nuclear and cytoplasmic extracts, respectively. (c) Proliferation index of BVECs and LVECs after overexpression of wt RhoB-Flag and its mutants at 24 h after proliferation challenge, determined as the ratio of the number of Ki67 positive cells to the total number of cells (expressed as %,n≥600 total cells taken from at least six fields with at least 100 cells per field per condition, mean±s.e.m., unpaired two-tailed Student’st-test). AdGFP was used as the control. (d) Relative levels of VEGF-R2 and NRP1 in BVECs, and TIMP3 in LVECs after overexpression of wt RhoB-Flag and its dominant negative mutant adRhoB-DN at 24 h after proliferation challenge as determined by QRT–PCR (mean±s.e.m., unpaired two-tailed Student’st–test). Figure 6: BVEC and LVEC proliferation is specifically regulated by GTP-bound state of RhoB. ( a ) Representative western blot for detection of RhoB protein activation by GTP pull-down assay after adenoviral-mediated overexpression of wt RhoB-Flag (adRhoB) and RhoB mutants, that is, adRhoB-DN for dominant negative (GDP-bound state), adRhoB-CA for constitutive active (GTP-bound state). AdGFP was used as the control. Anti-RhoB and anti-Flag antibodies successfully detected all RhoB-Flag proteins in input samples. ( b ) Representative western blot of nuclear and cytoplasmic extracts from BVECs and LVECs showing the dual localization of overexpressed wt RhoB-Flag and its mutants in both nuclei and cytoplasm of BVECs and LVECs. AdGFP was used as the control. DNA Polβ and Tubulin proteins were used as internal controls for nuclear and cytoplasmic extracts, respectively. ( c ) Proliferation index of BVECs and LVECs after overexpression of wt RhoB-Flag and its mutants at 24 h after proliferation challenge, determined as the ratio of the number of Ki67 positive cells to the total number of cells (expressed as %, n ≥600 total cells taken from at least six fields with at least 100 cells per field per condition, mean±s.e.m., unpaired two-tailed Student’s t -test). AdGFP was used as the control. ( d ) Relative levels of VEGF-R2 and NRP1 in BVECs, and TIMP3 in LVECs after overexpression of wt RhoB-Flag and its dominant negative mutant adRhoB-DN at 24 h after proliferation challenge as determined by QRT–PCR (mean±s.e.m., unpaired two-tailed Student’s t –test). Full size image To determine the biological effect of the GTP-bound versus the GDP-bound form of RhoB, we measured the proliferative index of BVECs and LVECs overexpressing either wt or mutant RhoB ( Fig. 6c ). As previously observed, wt RhoB promotes and represses the proliferation of BVECs versus LVECs, respectively. Interestingly, whereas RhoB-DN did not affect the proliferation rate of either type of endothelial cell, RhoB-CA influenced the proliferation of BVECs and LVECs similarly to wt RhoB. The lack of effect on proliferation by the RhoB-DN correlates with its inability to regulate genes previously identified as RhoB-VEZF1 targets such as VEGF-R2, NRP1 and TIMP3 ( Fig. 6d ). Altogether, these results suggest that both forms of RhoB may exist as part of the nuclear RhoB–VEZF1 transcriptional complex. However, only RhoB-GTP has the ability to regulate the expression of genes that are specific targets of RhoB–VEZF1 and modulate the proliferation rate of BVECs and LVECs. Targeting VEZF1 normalizes pathological angiogenesis in OIR Findings presented in Figs 1a and 4a suggest that RhoB in collaboration with VEZF1 promotes pathological angiogenesis accompanying OIR. We hypothesized that by interfering with the RhoB–VEZF1 pathway we might restore physiological revascularization in this setting. To target the RhoB–VEZF1–DNA complex we focused on the DNA-binding domain of VEZF1 composed of a zinc finger domain designed to recognize a specific DNA promoter sequence [32] . C2H2 zinc fingers occur in tandem arrays with many transcription factors composed of three or more fingers working in concert to bind its appropriate promoter [33] , [34] . Using an in silico approach we identified a small molecule that could inhibit the interaction of VEZF1 with DNA (D.S. ; personal communication). This structurally unique drug-like small molecule inhibitor of VEZF1 (VEC6; NSC 11435; two-dimensonal (2D) structure in Supplementary Fig. S5 ) significantly repressed NRP1 promoter-dependent luciferase activity in the presence of RhoB and VEZF1 overexpression ( Fig. 7a ). To further validate the efficacy of this compound, the expression pattern of several target genes downstream of RhoB and VEZF1 was evaluated in BVECs and LVECs undergoing proliferative stress in the absence or presence of VEC6 ( Fig. 7b ). This inhibitor repressed the expression of VEGF-R2, NRP1 and TIMP3 as determined by QRT–PCR. Interestingly, VEC6 phenocopies the opposing effects of RhoB-VEZF1, that is, it represses the proliferation of BVECs, and promotes the proliferation of LVECs ( Fig. 7c ). Importantly, these data provide additional support that VEC6 is working ‘on target’ to effectively modulate the RhoB–VEZF1–DNA complex. To evaluate the efficacy of this compound in vivo , neonatal RhoB +/− mice were subjected to the OIR assay in the presence of VEC6 or DMSO (vehicle), administered during the pathological phase (P12–P17) ( Fig. 7d ). Pups treated with DMSO showed no change in their pathological angiogenic response (compare Fig. 7d ). However, VEC6 treatment increased the emergence of blood vessels with a normal morphology (arrowheads), and reduced both the avascular areas and pathological glomeruloid bodies (more than twofold decrease in the number of nuclei interior to ILM). These data indicate that the VEZF1 inhibitor, VEC6, can modulate the activity of the RhoB–VEZF1 complex by disrupting the VEZF1–DNA interaction interface similar to the loss of RhoB. 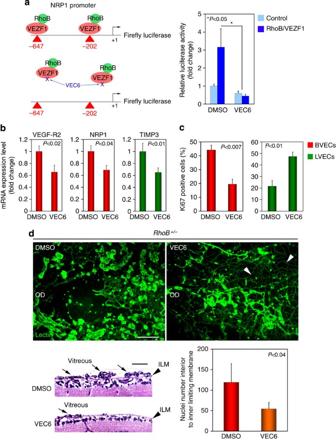Figure 7: Targeting VEZF1/DNA binding normalizes pathological angiogenesis during OIR. (a) Schematic drawings of the human NRP1 promoter containing predictedin silicoVEZF1 DNA binding sites (red triangles) depicting VEZF1 (red oval) binding to DNA, and RhoB (green circle) binding to VEZF1. The start site of transcription is referred as +1. The small molecule NSC 11435, named compound VEC6, shown docking to this VEZF1 zinc finger pocket (indicated by blue crosses) was screened for its ability to interfere with the interaction between VEZF1 and its DNA binding site leading to decreased promoter transactivation by the RhoB-VEZF1 complex. Activity of the human NRP1 promoter in Hela cells (control) and Hela cells overexpressing RhoB and VEZF1 (RhoB/VEZF1) in presence of solvent (DMSO) or VEC6 (20 nM for 24 h) (three independent experiments, each containing duplicates, mean±s.e.m., unpaired two-tailed Student’st-test). (b) Relative levels of VEGF-R2, NRP1, TIMP3 in BVECs and LVECs following treatment with compound VEC6 (20 nM for 24 h) as determined by QRT–PCR (mean±s.e.m., unpaired two-tailed Student’st-test). (c) Proliferation index of BVECs and LVECs treated with compound VEC6 at 24 h after proliferative challenge, determined as the ratio of the number of Ki67-positive cells to the total number of cells (expressed as %,n≥600 total cells taken from at least six fields with at least 100 cells per field per condition, mean±s.e.m., unpaired two-tailed Student’st-test). (d) Whole-mount staining of blood vessels (BS-I lectin) in the retina ofRhoB+/−pups subjected to OIR and treated with vehicle (DMSO) or compound VEC6 by daily intraperitoneal injection between P12 and P17 (OD=optic disc). Histological analysis (H&E staining) ofRhoB+/−retinas at P17 following treatment with DMSO or VEC6. Quantification of the number of nuclei interior to ILM (eight animals per group, mean±s.e.m., unpaired two-tailed Student’st-test). Scale bars: Whole-mount staining=100 μm, H&E sections=50 μm (d). Figure 7: Targeting VEZF1/DNA binding normalizes pathological angiogenesis during OIR. ( a ) Schematic drawings of the human NRP1 promoter containing predicted in silico VEZF1 DNA binding sites (red triangles) depicting VEZF1 (red oval) binding to DNA, and RhoB (green circle) binding to VEZF1. The start site of transcription is referred as +1. The small molecule NSC 11435, named compound VEC6, shown docking to this VEZF1 zinc finger pocket (indicated by blue crosses) was screened for its ability to interfere with the interaction between VEZF1 and its DNA binding site leading to decreased promoter transactivation by the RhoB-VEZF1 complex. Activity of the human NRP1 promoter in Hela cells (control) and Hela cells overexpressing RhoB and VEZF1 (RhoB/VEZF1) in presence of solvent (DMSO) or VEC6 (20 nM for 24 h) (three independent experiments, each containing duplicates, mean±s.e.m., unpaired two-tailed Student’s t -test). ( b ) Relative levels of VEGF-R2, NRP1, TIMP3 in BVECs and LVECs following treatment with compound VEC6 (20 nM for 24 h) as determined by QRT–PCR (mean±s.e.m., unpaired two-tailed Student’s t -test). ( c ) Proliferation index of BVECs and LVECs treated with compound VEC6 at 24 h after proliferative challenge, determined as the ratio of the number of Ki67-positive cells to the total number of cells (expressed as %, n ≥600 total cells taken from at least six fields with at least 100 cells per field per condition, mean±s.e.m., unpaired two-tailed Student’s t -test). ( d ) Whole-mount staining of blood vessels (BS-I lectin) in the retina of RhoB +/− pups subjected to OIR and treated with vehicle (DMSO) or compound VEC6 by daily intraperitoneal injection between P12 and P17 (OD=optic disc). Histological analysis (H&E staining) of RhoB +/− retinas at P17 following treatment with DMSO or VEC6. Quantification of the number of nuclei interior to ILM (eight animals per group, mean±s.e.m., unpaired two-tailed Student’s t -test). Scale bars: Whole-mount staining=100 μm, H&E sections=50 μm ( d ). Full size image Loss of RhoB decreased the extent of pathological angiogenesis in the ischaemic retina and led to a reduction in angiogenesis in response to dermal wounding, but unexpectedly enhanced lymphangiogenesis following both dermal wounding and inflammatory challenge. Although RhoB is induced in both BVECs and LVECs subjected to proliferative stress, RhoB promotes proliferation and sprouting in BVECs, but represses these functions in LVECs. We investigated the importance of a direct interaction between RhoB and the transcription factor VEZF1 in both BVECs and LVECs, and demonstrated that the GTP-bound form of RhoB found in the nucleus exclusively regulates VEZF1-mediated transcription of unique and relevant target genes in BVECs versus LVECs. We propose that this differential regulation is responsible, at least in part, for the well-documented phenomenon of delayed lymphangiogenesis observed in pathological settings in vivo [3] , [4] , [25] . VEZF1 encodes a zinc finger transcription factor essential for developmental angiogenesis and lymphangiogenesis. VEZF1 −/− embryos exhibit vascular remodelling defects, loss of vascular integrity, internal bleeding and embryonic death. Haploinsufficiency is observed in 20% of VEZF1 +/− embryos, resulting in lymphatic hypervascularity, oedema and haemorrhage [22] . Our present work provides further evidence for the cooperation of RhoB and VEZF1, particularly in the adult. To our knowledge, this is the first demonstration of a protein complex, that is, RhoB–VEZF1, which serves intra-cellular and opposing regulatory roles in two closely related endothelial cell types ( Fig. 8a ). 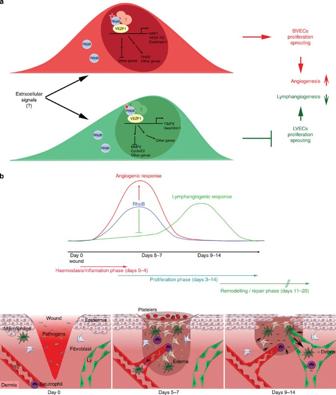Figure 8: Model for RhoB-mediated coordination of angiogenesis and lymphangiogenesis in dermal wounds. (a) After tissue challenge initiated by dermal wounding and in response to numerous extracellular signals that remain to be exploredin vivo, the immediate early response geneRhoBis induced and its protein accumulates in both blood and lymphatic vascular endothelial cells. The GTP-bound form of RhoB (red star) partially localizes in the nucleus of both cell types, where its physical interaction within the VEZF1 transcriptional complex regulates the differential expression of specific direct target genes in BVECs and LVECs leading to an increase in BVEC proliferation and sprouting and a simultaneous decrease in LVEC proliferation and sprouting. Accordingly, RhoB null mice exhibit reduced angiogenesis versus earlier, augmented and abnormal lymphangiogenesis in this and other pathological scenarios. (b) We propose that the opposing roles served by RhoB in these two endothelial cell types contribute to the coordination of an early angiogenic response versus a delayed lymphangiogenic response previously observed in wound healing. In this setting, the early angiogenic response participates in the initial inflammatory phase by facilitating recruitment of inflammatory cells into the wound bed (day 5–7). The delayed lymphangiogenesis allows these cells time to initiate tissue repair. Thereafter, the new lymphatics support the resolution of the local oedema (small black arrows) by draining fluid excess, cells and debris (big black arrow) (day 9–14). Figure 8: Model for RhoB-mediated coordination of angiogenesis and lymphangiogenesis in dermal wounds. ( a ) After tissue challenge initiated by dermal wounding and in response to numerous extracellular signals that remain to be explored in vivo , the immediate early response gene RhoB is induced and its protein accumulates in both blood and lymphatic vascular endothelial cells. The GTP-bound form of RhoB (red star) partially localizes in the nucleus of both cell types, where its physical interaction within the VEZF1 transcriptional complex regulates the differential expression of specific direct target genes in BVECs and LVECs leading to an increase in BVEC proliferation and sprouting and a simultaneous decrease in LVEC proliferation and sprouting. Accordingly, RhoB null mice exhibit reduced angiogenesis versus earlier, augmented and abnormal lymphangiogenesis in this and other pathological scenarios. ( b ) We propose that the opposing roles served by RhoB in these two endothelial cell types contribute to the coordination of an early angiogenic response versus a delayed lymphangiogenic response previously observed in wound healing. In this setting, the early angiogenic response participates in the initial inflammatory phase by facilitating recruitment of inflammatory cells into the wound bed (day 5–7). The delayed lymphangiogenesis allows these cells time to initiate tissue repair. Thereafter, the new lymphatics support the resolution of the local oedema (small black arrows) by draining fluid excess, cells and debris (big black arrow) (day 9–14). Full size image In particular, our work highlights the importance of the RhoB–VEZF1 pathway in the temporal regulation of angiogenesis and lymphangiogenesis during wound healing. Tissue damage (for example, skin wounds) triggers a healing response precisely coordinated through different phases, that is, haemostasis/inflammation, proliferation and remodelling/repair ( Fig. 8b ). The early pro-angiogenic response participates in the initial inflammatory phase by facilitating recruitment of inflammatory cells into the wound bed ( Supplementary Movie 8 ). Thereafter, the formation of local oedema enhances the migration of inflammatory cells, endothelial cells and myofibroblasts through the loose fibrin-rich provisional matrix of the granulation tissue to begin wound repair. Subsequently, the formation of new lymphatics aids in the drainage of excess fluid, cells and debris, to allow the remodelling phase to proceed, ultimately resulting in wound closure. Thus, RhoB, by its interaction with VEZF1, actively participates in ensuring the delay in lymphangiogenesis that appears to be crucial to the success of the overall wound-healing programme. Among the direct target genes of RhoB–VEZF1 pathway that we identified in BVECs, both VEGF-R2 and NRP1 are known to support angiogenesis elicited by the pro-angiogenic cytokine VEGF-A. The downregulation of these two receptors in the absence of RhoB would be expected to impair angiogenesis in response to pathological challenge, in agreement with our in vivo observations of decreased angiogenesis in two different tissues. Another gene that is downregulated in BVECS after silencing either RhoB or VEZF1 is the prolyl hydroxylase domain-2 protein, PHD2. PHD2 has been shown to be involved in normalization of tumour vascular network [35] . Haplodeficiency of PHD2 also redirects the specification of endothelial tip cells to a more quiescent cell type, lacking filopodia [35] and this could contribute to the normalization of the pathological vascular phenotype that we observed it the OIR model. Of the set of specific target genes that we identified in LVECs, MMP2 has already been linked with lymphatic sprouting [36] , but two other genes, that is, TIMP3 and Vasohibin1, have not historically been implicated in LVEC biology. However, recent data implicate Vasohibin1 in the inhibition of lymphangiogenesis and metastasis, supporting a potential correlation with the abnormal lymphatic phenotype (vessel enlargement and leakage) observed in our mice [37] . Thus, our study provides important new information to the growing list of genes specific to the blood versus lymphatic vasculature. Although we were unable to evaluate the impact of the RhoB–VEZF1 pathway on wound closure in the ear model, our parallel study of dorsal skin excisional wound healing revealed that healthy RhoB −/− mice did not exhibit any significant difference in the time required for complete wound closure as compared with wt mice [38] . This result correlates with previous work, that is, earlier and increased lymphangiogenesis elicited by VEGF-A overexpression did not affect the time required for wound closure in healthy animals [6] . In contrast, VEGF-C overexpression accelerated wound closure by inducing angiogenesis, lymphangiogenesis and recruitment of inflammatory cells in diabetic animals [9] . We recently observed a similar phenomenon in RhoB −/− diabetic mice [38] , suggesting that the impact of deregulation of angiogenesis and/or lymphangiogenesis by loss of RhoB could be exacerbated in pathological conditions such as those occurring in diabetic animals. Rho family GTPases control many different biological processes including cell survival, proliferation, adhesion, migration, gene expression and apoptosis [39] , and subcellular localization has been identified as a critical factor in the ability of these GTPases to function in different signalling pathways [40] . To date there have been only a few reports linking a Rho family GTPase found in the nucleus to the regulation of gene expression by a transcription factor. Both RhoA and Rac1 have been reported to participate in transcriptional complexes involving the transcription factors Glucocorticoid Receptors and beta-catenin/TCF4, respectively [41] , [42] . A recent study has reported a functional Net1/RhoA signalling pathway within the nucleus implicated in the DNA damage response [43] , and Rac1 signalling has also been shown to modulate a STAT5/BCL-6 transcriptional switch on cell-cycle-associated target gene promoters [44] . The nuclear localization of these small GTPases may be cell-type-specific, as we did not observe RhoA in the nucleus of BVECs and LVECs. However, our own findings provide strong evidence for the participation of nuclear RhoB–GTP in the efficient gene transcription by VEZF1 through their direct interaction in endothelial cell nuclei. The association of small GTPases with transcription factors in the nucleus is a relatively new finding; therefore, many outstanding questions remain to be addressed including the function served by the GTPase in the transcriptional complex, and the identity of additional proteins that participate in this transcriptional complex. It has been shown that the p68RacGAP interacts with VEZF1 and facilitates the hydrolysis of the GTP form of Rac1 in endothelial cells [45] . Future studies will be needed to identify the regulatory partners, for example, the GAPs and GEFs, present in the RhoB–VEZF1 transcriptional complex, that participate in the RhoB regulation of VEZF1-mediated gene transcription in BVECs versus LVECs. Finally, using an in silico approach we identified a small molecule inhibitor (VEC6) targeting the VEZF1–DNA binding interface that was able to recapitulate the effects of the loss of RhoB in the ischaemic retina. This finding suggests that the RhoB–VEZF1 complex represents an interesting new target for developing novel therapies against numerous pathologies with a vascular component, for example, diabetic retinopathy. However, VEC6 was also able to induce LVEC proliferation in vitro similar to silencing of RhoB , suggesting the possibility of a pro-lymphangiogenic effect in vivo . Further work using a second generation of inhibitory molecules more suited for in vivo studies in adult mice will be needed to address the question of lymphatic sensitivity and responsiveness. In conclusion, we propose that RhoB, an immediate early gene product, located in the nucleus in its GTP form, interacts with the transcription factor VEZF1 to drive transcription of unique target gene sets in BVECs versus LVECs, which in turn regulate, at least in part, the distinct blood and lymphatic endothelial responses to different pathological stimuli. Additional analysis of this transcriptional complex will further our understanding of its differential angiogenic and lymphangiogenic regulatory mechanisms and identify new therapeutic strategies for more specific intervention of the blood versus lymphatic vasculature. Our findings emphasize the broader worth of considering the potential impact on the lymphatic vascular network of any pro- or anti-angiogenic therapy. Further understanding the RhoB–VEZF1 pathway may provide crucial information relevant to the challenge of defining therapies that focus on one vascular bed versus the other, thus enlarging the impact of our study on the whole vascular field. Mice RhoB −/− mice, a gift from George Prendergast [19] , were maintained in both SV129 and FVB backgrounds. VEZF1 +/− mice, a gift from Heidi Stuhlmann [22] were maintained in the SV129 background. To study the functional cooperation between RhoB and VEZF1 in vivo , RhoB −/− mice in the SV129 background were crossed with VEZF1 +/− mice in the SV129 background. Resulting double heterozygotes were crossed to obtain all required genotypes in one litter ( RhoB +/− , VEZF1 +/− and RhoB +/− VEZF1 +/− ). All studies were conducted in compliance with the Beth Israel Deaconess Medical Center IACUC guidelines. Retinopathy of prematurity Neonatal mice (female and male, eight groups; five to six pups per group) were exposed to 75% oxygen beginning on post-natal day P7, and returned to room air on day P12. Retinas were harvested on day P17, fixed in 10% formalin for 1 h, and incubated with FITC-Lectin BS-1 (Sigma, St Louis, MO, USA) in PBS, 0.2% Triton X-100 and 10% Goat serum O/N at 4 °C. Retinas were washed (four to five times for 1 h) in PBS, flattened and photographed using a Leica MZFIII microscope and DC200 digital camera. Pups used to evaluate VEZF1 inhibitors were injected i.p. with 30 mg per kg per day of test compound from P12 to P17. Their retinas were processed and imaged as above. Ear acute injury and chronic inflammation Full-thickness wounds were created in the center of the ears of adult mice (female and male, 6–8 weeks) using a 2-mm biopsy punch. Seven days post-injury ears were examined by whole-mount staining and/or by intravital microscopy to assess both angiogenesis and lymphangiogenesis. Chronic inflammation was induced by DTH in the ear skin of RhoB null and wt mice as described previously [26] . Briefly, adult mice (6–8 weeks) were sensitized by topical application of a 2% oxazolone (4-ethoxymethylene-2 phenyl-2-oxazoline-5-one; Sigma) solution in acetone/olive oil (4:1 vol/vol) to the shaved abdomen (50 μl) and to each paw (5 μl). Five days later, ears were challenged by topical application of 1% oxazolone solution (20 μl). Ear swelling was assessed daily by ear thickness measurement using a Mitutoyo caliper for 11 days post-challenge. Lymphangiogenesis was assessed by intravital microscopy. Ear whole-mount staining Whole mounts of ears were prepared for confocal microscopy as previously described [8] . Ears from adult mice (female and male, 6–8 weeks) were dissected, split into the dorsal and ventral surface and fixed for 3 h in 4% PFA. Tissues were blocked overnight in PBS, 5% goat serum, 0.3% Triton X-100 and then incubated successively O/N in primary antibodies (CD31 (MEC13.3, 553370, BD Pharmingen), and Podoplanin (ab11936, Abcam)) and secondary antibodies (Jackson) each diluted 1/200 in blocking solution. Samples mounted on glass slides were observed with a confocal microscope (Zeiss LSM 510 Meta). Confocal 3D projections were processed by Zeiss LSM Image software. Each 3D projection image corresponds to a tissue thickness of 100 μm. CD31 signal of 3D projections was quantified by using the measure function (% Area) from NIH ImageJ software, after selection of the wound angiogenic area (white lines). Ear intravital microlymphangiography Microlymphangiography was performed as described [27] . Ears of anesthetized adult mice (female and male, 6–8 weeks) were mounted flat on a resin support, held in place by silicone vacuum grease and viewed in a Leica MZFLIII fluorescent microscope. FITC–dextran (2,000 kDa lysine-fixable, Invitrogen at 20 μg μl −1 in saline) was injected into the lymphatics through a 10-μm pre-pulled borosilicate glass micropipette (World Precision Instruments, Sarasota, FL, USA) attached to a 500 μl Hamilton syringe fitted with a threaded plunger. Using a micromanipulator (WPI), the micropipette was injected into the dorsal surface of the periphery of the ear in order to engage a lymphatic lumen. Additional tracer (5–20 μl) was then slowly injected under the control of a threaded plunger. The progress of the fluorescent tracer through the lymphatic network was followed in real time by digital image capture (60 frames min −1 ) using a Leica DC350 FX digital camera in conjunction with Image-Pro Plus 6.2 Software. The resultant image stack was combined to produce a movie of tracer transport. Isolated frames, corresponding to specific times following tracer injection, were used to quantify the FITC–dextran tracer signal in each image using the measure function (% area) from NIH ImageJ software. Human dermal microvascular endothelial cell isolation Primary dermal human microvascular endothelial cells (HMVECs) from human male foreskins (from at least four individuals) were isolated as previously described [46] . The Beth Israel Deaconess Medical Center IRB approved the use of this discarded tissue. No clinical information or method of identification of the donor is provided. Both BVECs and LVECs were isolated with magnetic Dynabeads pre-associated with CD31 (Invitrogen). Subsequently, LVECs were separated from BVECs by using goat anti-mouse Dynabeads associated with Podoplanin antibody (Angiobio). The purity of these two endothelial cell populations was assessed by Dil-Ac-LDL, CD31 and Prox1 staining ( Supplementary Fig. S2a ). A total of six different cell isolation lots were used at passages 4–5 for all in vitro experiments. Each experiment was performed on at least two different cell isolation lots. HMVECs were grown in pre-coated plates with collagen I in MCDB131 medium (CellGro) supplemented with L-Alanyl-L-Glutamine (CellGro, 2 mM) and MVGS (Cascade Biologics). Transfection siRNA transfection in HMVECs was performed using HMVEC-L Nucleofector kit (Lonza). Confluent cells were harvested with trypsin-EDTA, washed in PBS and added to nucleofection solution (100 μl per 1 × 10 6 cells). Programme S-005 was used for transfection. Cells were removed from the cuvette and plated into a pre-coated six-well culture plate. Final siRNA concentration was 50 μM in the plate. RhoB and VEZF1 were silenced by using pre-designed siRNAs from Ambion (RhoB: siRNA ID# 42060, 41981, 41889, and VEZF1: siRNA ID# S15222, S15223, S15224). Silencer Select Negative Control #1 siRNA served as control. VEZF1 overexpression was obtained by transfection of human VEZF1 expression vector (Origene). Luciferase assays were performed using the Dual-Luciferase Reporter Assay System (Promega). Adenovirus and mutagenesis RhoB-Flag adenoviruses were generated using AdEasy Adenoviral system (Promega). Briefly, human RhoB coding sequence was amplified from human primary endothelial cell cDNA and inserted in pShuttle-IRES-hrGFP-1. Site-directed mutagenesis of RhoB was induced by PCR using Phusion High-Fidelity DNA polymerase (Fynnzymes) and Dpn I digestion. Mutagenic primers were used to prepare mutants for Constitutive Active (G14V) and Dominant Negative (T19N) forms of RhoB. All wt and mutant sequences were checked by DNA sequencing. AdEasy recombinants were generated by electroporation of BJ5183 cells containing pAdEasy-1 vector, with Pme I linearized shuttle vector. Adenoviruses were expanded in 293FT cells and purified with two CsCl centrifugations. Purified adenoviruses were stored in Viral Preservation Media (Tris–HCl 20 mM pH 8, MgCl 2 2 mM, sucrose 5%) at −80 °C. Cells were infected at an MOI of 50 pfu per cell. Cell immunostaining Human dermal endothelial cells, grown in complete medium on coverslips pre-coated with collagen, were collected after 24 h to assess the proliferation rate with Ki67 antibody (18-0191Z, ZYMED) or at confluence for Prox1 (20R-PR039, Fitzgerald) and CD31 (555444, BD Pharmingen) immunostaining to confirm BVECs versus LVECs population identity. Cells were fixed with 4% paraformaldehyde for 5 min, permeabilized and blocked with PBS, 5% goat serum, 0.1% Triton X-100 for 1 h at room temperature. Primary antibodies were diluted 1/200 in blocking solution without Triton X-100 and then incubated with cells at 4 °C O/N followed by appropriate secondary antibody (Jackson). Coverslips were washed and mounted in Dako Fluorescent Mounting Medium containing DAPI (3 μg ml −1 ). Quantification of the proliferation rate with Ki67 antibody was determined by the analysis of three independent experiments and 10 random fields for each experiment. Sprouting assay Spheroid production was performed as described [47] . In 96-well plates, 400 endothelial cells per well were seeded in 100 μl per well of MVGS media containing 20% Methylcellulose (Sigma). After 24 h, cell aggregates, named spheroids, were collected and centrifuged. Three-dimensional cultures of spheroids were prepared by using the overlay method as previously described [48] . Spheroids were resuspended in media containing 2% Growth factor-reduced Matrigel (BD Biosciences), and seeded on top of the underlay containing a 50:50 mixture Matrigel and Bovine collagen I (PureCol, 3 mg ml −1 , Inamed Biomaterials). Before mixing, collagen I was neutralized by addition NaOH (10 mM) in 1 × PBS and the pH was brought to 7.5 by using 0.1 M HCl. Stimulatory cytokine, (human VEGF-A (25 ng ml −1 ) or human VEGF-C (100 ng ml −1 ) (RD Systems), respectively for BVECs and LVECs) was added to the Matrigel/collagen I underlay mixture. After 24 h of stimulation, phase-contrast pictures were taken using a microscope (Nikon eclipse TE300) equipped with a camera (Leica, DFC 350 FX). Fluorescent images of GFP-positive cells were obtained by confocal microscopy (Zeiss LSM 510 Meta). For quantification, the cumulative sprout length of 15 randomly selected spheroids from three independent experiments was reported per data point. Cell extracts and immunoblot analysis Cytoplasmic extracts were obtained by using a cytoplasmic lysis buffer (Triton X-100 0.25%, Tris–HCl 10 mM (pH 8), EDTA 5 mM, EGTA 0.5 mM and proteases inhibitors (Sigma-P8340)). After centrifugation, the nuclei pellet was resuspended in Urea lysis buffer (Urea 8 M, Tris–HCl 50 mM pH 8, EDTA 5 mM and proteases inhibitors). Total extracts were formed by direct cell digestion in urea lysis buffer. Western blot analysis was performed as described [49] . Briefly, total extracts were separated on SDS–PAGE and membranes probed with antibodies recognizing human RhoB (1 in 500) (Cell Signaling-2098), RhoA (1 in 500) (Bethyl-lab-929), VEZF1 (1 in 500) (Abcam-ab50970), Tubulin (1 in 1,000) (Calbiochem-CP06), DNA polymerase β (1 in 500) (Abcam-26343), LYVE-1 (1 in 500) (UpState-07-538), Prox1 (1 in 500) (Fitzgerald-20R-PR039), CD31 (1 in 500) (BDPharmingen-555444), Podoplanin (1 in 500) (Angiobio-11-003), VEGFR3 (1 in 500) (SantaCruz-sc-321) and Flag tag (1 in 500) (Abcam-ab1162). Chromatin immunoprecipitation ChIPs were performed using 0.5 × 10 6 cells per IP. Proteins were first crosslinked with 1.5 mM EGS [50] , and were then crosslinked to DNA with 1% formaldehyde. After cytoplasmic fractionation, nuclei were digested in Complete Digestion Buffer from Nuclear complex Co-IP kit (Active motif). DNA was sheared by sonication. IP protocol was followed as described by supplier. Each IP was performed using 6 μg of antibodies against human VEZF1 (Abcam-ab85414), Flag tag (Sigma-F1804) and human Polymerase II (Covance-MMS-126R) and compared with IgG controls. DNA was purified as described in (ref. 51 ). Briefly, formaldehyde crosslinks were reversed at 67 °C for overnight. Samples were incubated with RNaseA and purified using Qiagen Qiaquick PCR purification kit. DNA enrichment was analysed by real-time PCR. GTP pull-down assay RhoB activity was assessed by measuring the amount of GTP-bound form of RhoB using the small GTPase activation assay (STA-403) from Cell Biolabs. In all, 5 × 10 6 cells were used for each pull-down reaction performed with Rhoketin RBD Agarose beads, as described by manufacturer. The proteins were revealed by immunoblot analysis using antibodies recognizing human RhoB and Flag tag. Analysis of gene expression Total RNAs from two independent cell isolation lots, each from at least four separate individuals, were isolated using RNeasy Kit and treated by DNase I during extraction steps (Qiagen). cDNAs were prepared from 0.5 μg total RNA using random hexaprimers as templates and SuperScript III (Invitrogen). Quantitative real-time RT–PCR (QRT–PCR) was carried out on an AbiPrism 7500 system using SYBR Green. The primer sequences are available in Supplementary Table S2 . For Affymetrix GeneChip probe array, 1 μg total RNA of one cell isolation lot from at least four separate individuals was used to synthetize cRNA, which was hybridized to Affymetrix HT Human U133A GeneChips. Fold change of gene expression and GO analysis were established using the dChip software [52] . Present probe sets with a differential expression of ≥1.5-fold and P <0.05 were taken into account. Proximity ligation assay Cells grown on collagen-coated 10-cm culture plates were co-transfected with 0.5 μg each of DNA encoding Flag-VEZF1 (OriGene) and V5-RhoB (HMVEC-L kit from Lonza). Cells were plated in collagen-coated eight-well slide chambers and incubated for 24 h at 37 °C to allow protein expression, then fixed, permeabilized and incubated with primary antibodies (mouse monoclonal anti-Flag (Sigma-F1804) plus rabbit polyclonal anti-V5 (Abcam-ab15828), all diluted 1:400) for 1 h. Cells were washed with provided blocking buffer and then incubated for 1 h with anti-mouse (+) and anti-rabbit (−) proximity ligation secondary antibodies, diluted 1:5, at 37 °C (PLA, DuolinkII system from Olink Bioscience). DNA amplification and fluorescent probes hybridization were performed as per instructions. Coverslips were mounted on slides and imaged by A1 Nikon confocal imaging system. Statistical analysis Results were presented as mean±s.e.m. Statistical significance of all data were analysed using the unpaired two-tailed Student’s t -test in the Microsoft Office Excel 2003 software. P -values <0.05 were considered to be statistically significant. Accession codes: Microarray data have been deposited in Gene expression omnibus under accession code GSE51754 . How to cite this article: Gerald, D. et al. RhoB controls coordination of adult angiogenesis and lymphangiogenesis following injury by regulating VEZF1-mediated transcription. Nat. Commun. 4:2824 doi: 10.1038/ncomms3824 (2013).